A comprehensive multiscale framework for simulating optogenetics in the heart Optogenetics has emerged as an alternative method for electrical control of the heart, where illumination is used to elicit a bioelectric response in tissue modified to express photosensitive proteins (opsins). This technology promises to enable evocation of spatiotemporally precise responses in targeted cells or tissues, thus creating new possibilities for safe and effective therapeutic approaches to ameliorate cardiac function. Here we present a comprehensive framework for multiscale modelling of cardiac optogenetics, allowing both mechanistic examination of optical control and exploration of potential therapeutic applications. The framework incorporates accurate representations of opsin channel kinetics and delivery modes, spatial distribution of photosensitive cells, and tissue illumination constraints, making possible the prediction of emergent behaviour resulting from interactions at sub-organ scales. We apply this framework to explore how optogenetic delivery characteristics determine energy requirements for optical stimulation and to identify cardiac structures that are potential pacemaking targets with low optical excitation thresholds. Electrical stimulation of the heart is a mainstay of modern cardiology, widely used for treating a range of heart rhythm disorders and for improving pump function. Direct current delivery from a lead in contact with the heart is used to evoke local excitation for pacemaking, cardiac resynchronization therapy and antitachycardia pacing; delivery of large currents by imposing strong electric fields (shocks) across the heart is used to elicit a global electrical response that terminates lethal arrhythmias. Despite this widespread and successful usage, the electrical stimulation paradigm is associated with numerous drawbacks. Pacing devices have limited autonomic responsiveness [1] ; electrochemical reactions at the electrode–tissue interface limit stimulus amplitude and duration [2] , and complications can arise during device implantation (infection) [3] or extraction (lead fracture) [4] . Moreover, paced ventricular excitation often results in an asynchronous activation sequence [5] , which is a poor substitute for normal sinus rhythm, leading to increased incidence of atrial fibrillation (AF), heart failure and death [6] . High-voltage cardioversion and defibrillation shocks have significant adverse consequences, including cellular electroporation [7] , disruption of normal cardiac electrical rhythm [8] and mechanical function [9] , increased mortality [10] , [11] , and psychological trauma [12] , leading to discontinuation of treatment [13] and increased procedure cost [14] . Optogenetics is an emerging field in which optical illumination is used to elicit a bioelectric response in excitable tissue that has been modified to express light-sensitive ion channel proteins called opsins [15] . Photon absorption triggers conformational changes in these proteins, allowing a transient flow of transmembrane current; photo-evoked current is potentiated by the energy content of incident light. Depending on which opsin is expressed, photo-evoked current can be depolarizing (inward) or hyperpolarizing (outward). Optical stimulation is envisioned to result in a broad range of applications because optogenetic schemes can selectively deliver light sensitivity to specific cell types using genetic promoters [16] or to specific functional regions [17] , as demonstrated in neuroscience. Moreover, as the energy transduction mechanism is fundamentally different from conventional electrical stimulation (transmembrane current as opposed to Faradaic charge transfer), the range of safe pulse widths and amplitudes is dramatically expanded for optical stimulation [18] . Once delivery techniques have been adapted and perfected to work effectively in the heart, optogenetics is expected to enable the evocation of precise spatiotemporal patterns of transmembrane current in any genetically targetable subpopulation of cardiac cells for which direct illumination is physically possible. As such, it is clear that optogenetics has the potential to transform the field of cardiac electrophysiology, rewriting the rules that govern the design of safe, effective and energy-efficient stimulation applications. Initial experiments attempting light-based stimulation of cardiac tissue have yielded exciting results [19] . Optical sensitivity has been inscribed in working heart cells in vitro using the photosensitive cation channel Chlamydomonas channelrhodopsin-2 (ChR2), either by direct gene delivery (GD) using viral vectors [20] or by cell delivery (CD), where cardiomyocytes are cocultured with (and coupled to) ChR2-rich inexcitable cells [21] . Experiments in transgenic mice have demonstrated the feasibility of optically pacing the mammalian heart in vitro and in vivo [22] . Cardiac electrophysiology and electromechanics modelling are recognized as vital tools for mechanistic enquiry, allowing researchers to test clinically relevant hypotheses at various scales of structural hierarchy, from the molecular to that of the entire organ [23] . Developing the ability to simulate cardiac optogenetics in a realistic manner within a biophysically detailed whole-heart modelling infrastructure is an essential step in the quest to obtain novel solutions for optical pacing, defibrillation and other types of electrophysiological control of cardiac behaviour. Tools for modelling cardiac optogenetics will accelerate the translation of this exciting technology to the clinic by providing an accurate and efficient platform for assessing the feasibility of potential optical control strategies. The first objective of this study is to develop a comprehensive but flexible framework for simulating cardiac optogenetics. To achieve this goal, we identify key properties of light sensitivity, as well as its inscription in tissue and actuation by light, which need to be incorporated in the simulation framework to ensure its broad usefulness and the accuracy of its solutions. We then describe how each of these properties are integrated within a multiscale simulation hierarchy for modelling cardiac function. The second objective of this study is to demonstrate the utility of the framework in simulating a set of illustrative examples of optogenetic applications. We investigate optical stimulation efficiencies in models with different opsin delivery modes and spatial distributions of light-sensitive cells and explore differential stimulation by cell-specific targeting. Finally, we showcase the modularity of the optogenetics simulation framework by demonstrating the ease with which it can be integrated with models of arbitrary complexity. 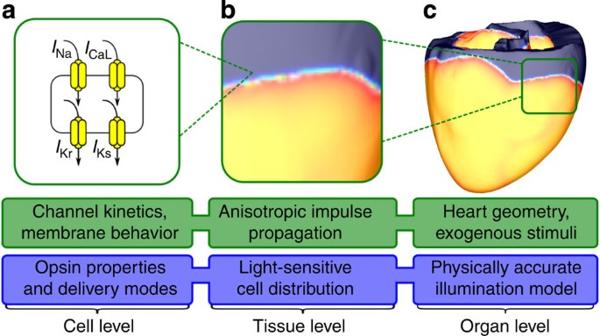Figure 1: New features for simulating optogenetics. Optogenetics simulation components (blue) are developed at each level of the existing multiscale cardiac model hierarchy (green). (a) Fundamental building blocks of our optogenetic modelling at the cell level include photo-evoked current in opsins and opsin delivery modes. We represent opsin currents as complex photokinetic processes that depend non-linearly on light, membrane voltage and time29. Opsins are either directly delivered to normal myocytes using viral vectors20(GD mode) or expressed in inexcitable donor cells (CD mode), which can form gap junctions with host myocytes21. (b) At the tissue level, our optogenetic simulation framework incorporates heterogeneous spatial distribution of light-sensitive cells; this is important because diffuse, patchy patterns have been observed for both transgene34and donor cell35distribution in the heart. (c) At the organ level, our framework accounts for practical limitations associated with illumination, namely the limited ability of light to penetrate tissue without significant attenuation due to energy absorption and photon scattering37. Overview of key optogenetic framework components Figure 1 presents a multiscale model hierarchy for cardiac electrophysiology simulations (description of modules’ function is in green). This type of hierarchy has been described and successfully applied in mechanistic studies of cardiac rhythm dysfunction and therapy by our group [24] , [25] and others [26] , [27] , [28] . To develop cardiac optogenetic simulation capabilities on the basis of this model hierarchy, we develop and introduce new model features at each spatial scale (cell, tissue and organ levels, see blue boxes), as described in detail in the following sections. The framework we have developed is capable of representing opsin delivery using gene or cell therapy approaches and incorporates realistic representations of spatial distribution of light-sensitive cells and in vivo illumination constraints. Figure 1: New features for simulating optogenetics. Optogenetics simulation components (blue) are developed at each level of the existing multiscale cardiac model hierarchy (green). ( a ) Fundamental building blocks of our optogenetic modelling at the cell level include photo-evoked current in opsins and opsin delivery modes. We represent opsin currents as complex photokinetic processes that depend non-linearly on light, membrane voltage and time [29] . Opsins are either directly delivered to normal myocytes using viral vectors [20] (GD mode) or expressed in inexcitable donor cells (CD mode), which can form gap junctions with host myocytes [21] . ( b ) At the tissue level, our optogenetic simulation framework incorporates heterogeneous spatial distribution of light-sensitive cells; this is important because diffuse, patchy patterns have been observed for both transgene [34] and donor cell [35] distribution in the heart. ( c ) At the organ level, our framework accounts for practical limitations associated with illumination, namely the limited ability of light to penetrate tissue without significant attenuation due to energy absorption and photon scattering [37] . Full size image Modelling ChR2 properties and delivery modes Current flow in cardiac tissue is driven by active processes of ionic exchange across myocyte membranes. In a mathematical framework, these processes are represented by the ionic model of myocyte membrane behaviour, where current flow through ion channels, pumps and exchangers and current resulting from subcellular calcium cycling are governed by a set of ordinary differential and algebraic equations. The sum of all these currents is denoted by I ion ; in our framework, cell-level optogenetic properties were represented by incorporating a light-sensitive component in I ion . Our model of ChR2-mediated current ( I ChR2 ) is built on a Markov model proposed by Nikolic et al. [29] , derived from a channelrhodopsin-1 description by Hegemann et al. [30] ( Fig. 2a ). We adjusted model parameters to better match experimental recordings of I ChR2 collected from a stable ChR2-expressing human embryonic kidney (HEK) cell line [21] ; full details of our I ChR2 model can be found in the Methods section. 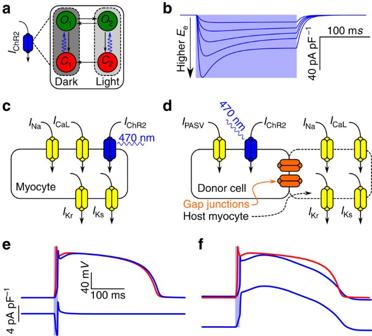Figure 2: Modelling ChR2 properties and delivery modes at the cell level. (a) Four-state Markov model forIChR2with dark- and light-adapted photocycle branches associated with different peak conductances; each branch comprises closed- (red) and open-channel (green) states. Channel opening rates (blue arrows) are directly proportional to the irradiance (Ee) of light absorbed by ChR2 and open channels approach anEe-dependent equilibrium between open statesO1andO2; all other transitions are purely time-dependent. (b)IChR2in response to illumination (pale blue background; top to bottom:Ee=0.4, 1, 2, 4 and 10 mW mm−2) withVmclamped to −85.6 mW. Photo-evoked ChR2 current has well-defined transient and steady-state phases resulting from the transition from full dark adaptation to an equilibrium between the two operating modes. TheIChR2model qualitatively reproduces experimental records from whole-cell patch-clamp recordings in a stable HEK-ChR2 cell line21, as shown inSupplementary Fig. S1. (c,d) Schematics for modelling gene delivery (GD) and cell delivery (CD) of ChR2; generic ionic currents are shown in myocytes. (e) Optically evoked (blue) and electrically evoked (red) APs and underlyingIChR2in a myocyte with gene-delivered ChR2. Illumination at 2 × threshold (Ee=0.468 mW mm−2over 10 ms) elicited depolarizingIChR2(bottom), which triggered an optically evoked AP. (f) Response to illumination in an inexcitable ChR2-rich donor cell (CD; dashed blue) coupled to a normal myocyte by a 500 MΩ resistance (solid blue); a photo-evoked AP in the latter cell is compared with an electrically evoked AP (red). Light delivered to the donor cell was at 2 × threshold for optically eliciting an AP in the myocyte (Ee=0.652 mW mm−2over 10 ms). During the AP plateau phase, myocyteVm(≈2.77 mV) was between the plateauVmof the electrically induced AP (≈15.3 mV) and the donor cell resting level (−40 mV). Figure 2b shows the irradiance-potentiated response of our I ChR2 model to illumination in a cell clamped to resting ventricular myocyte membrane voltage ( V m ). Figure 2: Modelling ChR2 properties and delivery modes at the cell level. ( a ) Four-state Markov model for I ChR2 with dark- and light-adapted photocycle branches associated with different peak conductances; each branch comprises closed- (red) and open-channel (green) states. Channel opening rates (blue arrows) are directly proportional to the irradiance ( E e ) of light absorbed by ChR2 and open channels approach an E e -dependent equilibrium between open states O 1 and O 2 ; all other transitions are purely time-dependent. ( b ) I ChR2 in response to illumination (pale blue background; top to bottom: E e =0.4, 1, 2, 4 and 10 mW mm −2 ) with V m clamped to −85.6 mW. Photo-evoked ChR2 current has well-defined transient and steady-state phases resulting from the transition from full dark adaptation to an equilibrium between the two operating modes. The I ChR2 model qualitatively reproduces experimental records from whole-cell patch-clamp recordings in a stable HEK-ChR2 cell line [21] , as shown in Supplementary Fig. S1 . ( c , d ) Schematics for modelling gene delivery (GD) and cell delivery (CD) of ChR2; generic ionic currents are shown in myocytes. ( e ) Optically evoked (blue) and electrically evoked (red) APs and underlying I ChR2 in a myocyte with gene-delivered ChR2. Illumination at 2 × threshold ( E e =0.468 mW mm −2 over 10 ms) elicited depolarizing I ChR2 (bottom), which triggered an optically evoked AP. ( f ) Response to illumination in an inexcitable ChR2-rich donor cell (CD; dashed blue) coupled to a normal myocyte by a 500 MΩ resistance (solid blue); a photo-evoked AP in the latter cell is compared with an electrically evoked AP (red). Light delivered to the donor cell was at 2 × threshold for optically eliciting an AP in the myocyte ( E e =0.652 mW mm −2 over 10 ms). During the AP plateau phase, myocyte V m (≈2.77 mV) was between the plateau V m of the electrically induced AP (≈15.3 mV) and the donor cell resting level (−40 mV). Full size image When light sensitivity is inscribed via GD, photo-evoked current directly affects excitable cells [20] , [22] . To represent this delivery mode in our framework, the I ChR2 model was added to I ion for species- and cell type-specific membrane models of ion kinetics ( Fig. 2c ), allowing simulation of species- and cell type-specific photo-evoked action potentials (APs). When light sensitivity is inscribed via CD, I ChR2 increases V m in ChR2-rich donor cells, establishing a potential gradient with coupled host myocytes; this gives rise to junctional currents, which depolarize host cells and evoke APs [21] . To represent membrane behaviour in light-sensitive donor cells I ion was replaced by I PASV , a model of electrically passive current with properties based on experimental measurements from HEK cells (used here as a model for donor cells; see Methods section), combined with the I ChR2 model. The resulting model of ChR2-expressing donor cell behaviour was either resistively coupled to a host myocyte model to simulate an optically excitable tandem pair ( Fig. 2d ) or integrated in a tissue-scale model to represent a syncytium of donor and host cells, as described in the next section. Figure 2e shows an optically evoked AP (top) in a human ventricular myocyte model [31] with ChR2 inscribed by GD; the AP in response to electrical stimulation in the same cell is superimposed for comparison. Differences between the optically and electrically evoked APs in the notch and plateau phases were due to non-instantaneous ChR2 channel closing kinetics. Figure 2f compares the same electrically induced AP to the response of a normal myocyte (top) resistively coupled ( R =500 MΩ) to an illuminated ChR2-rich donor cell (CD; bottom). Initial donor cell depolarization elicited myocyte depolarization via junctional current, leading to an AP. Following the myocyte upstroke, electrotonic coupling resulted in a plateau phase in both cells. The characteristics observed here qualitatively resembled the experimentally observed response to optical stimulation in tandem preparations of ChR2-rich HEK cells and myocytes [21] . Modelling spatial distribution of light-sensitive cells At the tissue level, AP propagation due to current flow between cells coupled by gap junctions is modelled by solving one or more partial differential equations [32] , [33] . Preferential conduction in the direction of myocardial fibres is incorporated via spatially varying anisotropic conductivity tensors. In vivo ChR2 delivery in whole hearts has not yet been reported, but observations from injection of non-optogenetic viral vectors [34] or donor cells [35] to the heart suggest that ChR2 delivery sites will comprise interdigitated clusters of light-sensitive cells and normal myocytes. This type of distribution has also been observed in cardiac cell monolayers with cell-delivered ChR2 [21] . Our framework modelled this heterogeneous distribution of light-sensitive cells within target sites of ChR2 delivery. To generate realistic spatial distributions of ChR2-expressing cells, we adapted a stochastic algorithm originally used to model fibrosis patterns in cardiac tissue [36] . For each ChR2 delivery target region, the parameters D and P controlled the density (by volume) and level of patchiness of light-sensitive cell clusters, respectively. Different parameter values resulted in a variety of stochastically generated distributions ( Fig. 3a–c ) consistent with experimentally observed patterns of transgene expression in mouse hearts [34] and aggregation of injected donor cells in dog hearts [35] . Full details of our implementation of this algorithm as well as a description of our approach to modelling electrical propagation in donor cell clusters can be found in the Methods section. 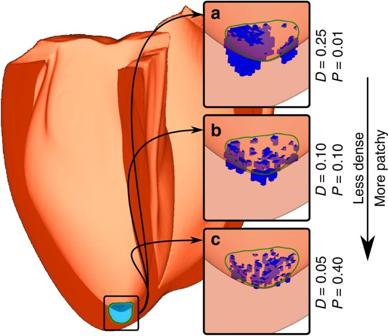Figure 3: Modelling spatial distribution of light-sensitive cells at the tissue level. Human ventricular model with a photosensitization target (green boundary; hemispherical, 1 cm diameter) near the LV apex. (a–c) Results of applying the light-sensitive cell distribution algorithm to populate the target region with framework-generated ChR2-expressing clusters (blue) for three combinations of the parametersD(density) andP(patchiness). Figure 3: Modelling spatial distribution of light-sensitive cells at the tissue level. Human ventricular model with a photosensitization target (green boundary; hemispherical, 1 cm diameter) near the LV apex. ( a – c ) Results of applying the light-sensitive cell distribution algorithm to populate the target region with framework-generated ChR2-expressing clusters (blue) for three combinations of the parameters D (density) and P (patchiness). Full size image Modelling light attenuation State-of-the-art cardiac models typically incorporate three-dimensional (3D) heart geometry and fibrous structure from various imaging modalities. For optogenetic applications, issues of light distribution and attenuation in the ventricular walls need to be considered at this scale [37] . Photo-evoked I ChR2 has an insignificant depolarizing effect unless the illumination source delivers blue light with a wavelength near 480 nm and with E e ≥0.1 mW mm −2 (ref. 29 ). We modelled optical stimulation with direct endocardial surface illumination with blue light, which is currently the only viable option for depolarizing photostimulation—efforts to red-shift excitatory opsins have had limited success [17] and two-photon excitation of ChR2, although possible [38] , is impractical outside laboratory settings. We assumed fixed irradiance values ( ) at endocardial surface points being illuminated and modelled attenuation in cells beneath the surface by , where r is the distance to the nearest site of direct illumination and δ is a wavelength-dependent decay coefficient. Previous simulations of cardiac optical mapping have proven that this formulation (with δ =570 μm) is an excellent model of depth-dependent attenuation in heart tissue uniformly illuminated by blue light near the range for ChR2 stimulation (488 nm) [39] . As shown by the spatial distributions of E e ( Fig. 4 ) resulting from uniform ( a ) or focal ( b ) illumination of the endocardium, only a thin (≈1.5 mm) layer of cells near the surface received an appreciable proportion of the energy in applied light. 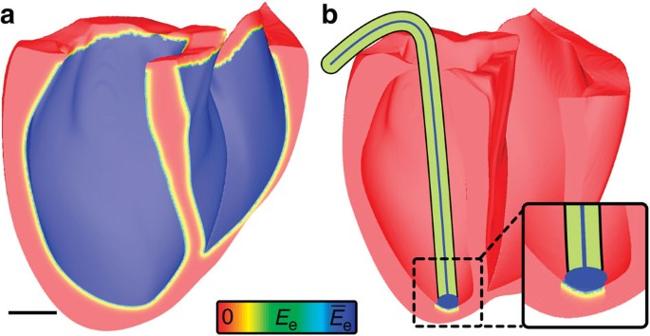Figure 4: Modelling light attenuation at the organ level. (a) Spatial profile of effectiveEe(normalized to surface irradiance) in human ventricular model with uniform illumination of the entire endocardium; scale bar, 20 mm. (b) The limited extent of illuminated tissue is emphasized for a more realistic illumination configuration, in which the tip of an optrode—an ensheathed bundle of optical fibres—was pressed against the endocardium and delivered unattenuated light to tissue directly below. Figure 4: Modelling light attenuation at the organ level. ( a ) Spatial profile of effective E e (normalized to surface irradiance ) in human ventricular model with uniform illumination of the entire endocardium; scale bar, 20 mm. ( b ) The limited extent of illuminated tissue is emphasized for a more realistic illumination configuration, in which the tip of an optrode—an ensheathed bundle of optical fibres—was pressed against the endocardium and delivered unattenuated light to tissue directly below. Full size image Optogenetic pacing of the human heart As experimental studies in cardiac optogenetics are presently in a gestational stage, it is unknown what opsin delivery schemes and illumination strategies are technologically feasible; our newly developed framework is a platform for simulating speculative scenarios that provide insight and guidance into future optogenetic developments. To demonstrate how insights can be gained by using our framework, we present illustrative examples of simulated cardiac optogenetics in two validated, biophysically detailed ventricular models [24] , [25] ; comprehensive model descriptions are provided in the Methods section. In the first illustrative example, we sought to examine optical stimulation efficiency for different optogenetic configurations (that is, combinations of ChR2 delivery mode and light-sensitive cell spatial distribution) in a magnetic resonance imaging-based model of the human ventricles [24] ; it is important to understand how these factors affect the energy required to stimulate optically because optogenetic techniques will need to be very efficient to be clinically viable and attractive as alternatives to conventional strategies. For the three light-sensitive cell spatial distributions shown in Fig. 3a–c for both CD and GD, optical stimulation was applied to the endocardial surface under the simulated optrode and efficiency was quantified by calculating the threshold irradiance required to elicit a propagating response ( E e,thr ). These three spatial distributions were chosen to represent different stages in the evolution of a ChR2 delivery site over time as transfected cells or donor cells die and migrate away from the injection site; the progression was from an initially dense, consolidated mass of light-sensitive cells (high D , low P ) to a sparse, patchy distribution (low D , high P ), as observed experimentally for GD [34] and CD [35] . 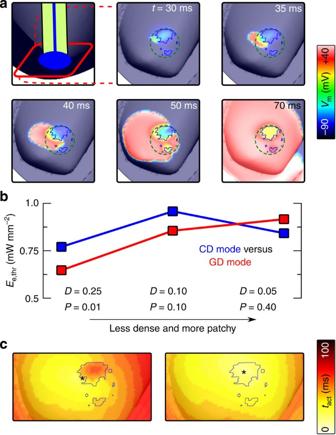Figure 5: Determinants of optical stimulation efficiency in the human ventricles. (a) Membrane voltage (Vm) response to 10 ms blue light pulse att=0. Cell-delivered ChR2 was distributed as inFig. 3a(D=0.25,P=0.01); blue outlines in zoomed-in panels indicate boundaries of ChR2-rich donor cell clusters. Optical stimulation just above threshold (Ee,thr=0.769 mW mm−2) was applied to the endocardial surface local to the ChR2 delivery site (dashed green line is contour of illuminated area).Supplementary Movie 1shows an animation of the full sequence. (b)Ee,thrvalues for all optogenetic delivery/distribution configurations. (c) Activation maps for CD mode (top) and GD mode (bottom) ChR2 in the same pattern as (a). Sites of earliest activation are marked by asterisks. Figure 5a shows the ventricular response to optical stimulation in a configuration with large, consolidated donor cell clusters. AP propagation initiated on the left-hand side of the delivery site, in a region of extensive interdigitation between ChR2-rich donor cells and myocytes; subsequently, activation spread towards the base of the heart. As summarized in Fig. 5b , the spatial distribution of light-sensitive cells affected E e,thr differently depending on ChR2 delivery mode. For GD of ChR2 in whole-heart models, as light-sensitive myocyte clusters became smaller and more sparsely distributed, optical stimulation efficiency decreased ( E e,thr rose monotonically); for CD mode, the least dense, patchiest ChR2-expressing donor cell patterns were associated with lower E e,thr values compared with distributions with intermediate D and P values. Figure 5: Determinants of optical stimulation efficiency in the human ventricles. ( a ) Membrane voltage ( V m ) response to 10 ms blue light pulse at t =0. Cell-delivered ChR2 was distributed as in Fig. 3a ( D =0.25, P =0.01); blue outlines in zoomed-in panels indicate boundaries of ChR2-rich donor cell clusters. Optical stimulation just above threshold ( E e,thr =0.769 mW mm −2 ) was applied to the endocardial surface local to the ChR2 delivery site (dashed green line is contour of illuminated area). Supplementary Movie 1 shows an animation of the full sequence. ( b ) E e,thr values for all optogenetic delivery/distribution configurations. ( c ) Activation maps for CD mode (top) and GD mode (bottom) ChR2 in the same pattern as ( a ). Sites of earliest activation are marked by asterisks. Full size image Delivery mode-dependent differences in tissue-level excitation mechanisms are explored in Fig. 5c . Activation maps for the response to illumination given CD (left) and GD (right) of ChR2 in the same consolidated spatial pattern (blue outline) reveal different sites of earliest propagation. For CD, initial excitation was on the boundary of the donor cell cluster, in an area of extensive interdigitation between ChR2-rich inexcitable cells and myocytes; the site of peak donor cell density was associated with delayed activation. For GD, the same site was colocalized with the earliest activation. Similar differences between the responses to illumination for CD and GD of ChR2 were observed in configurations with different spatial distributions. This explained why E e,thr was lower for CD compared with GD when D was low and P was high ( Fig. 5b , right side)—compared with other parameter combinations, these spatial distributions had the lowest peak local density of ChR2-expressing cells and the highest peak local contact area between light-sensitive cell clusters and normal myocardium; in other words, these distributions maximized the amount of interface between electrical sources and sinks during illumination. Thus, when donor cell or viral vector delivery of ChR2 to the intact heart results in light-sensitive cells distributed in small, patchy clusters—as observed for non-optogenetic cardiac cell and gene therapy injections [34] , [35] —our model predicts that optical stimulation efficiency will be higher for CD compared to GD. This demonstrates how our framework will help guide the development of efficient ChR2 delivery strategies as experiments in cardiac optogenetics move from light-sensitive tissue culture and transgenic animal models to in vivo applications. Targeted optogenetic stimulation of specialized tissue In the second illustrative example, we sought to compare optical stimulation efficiency in models with GD of ChR2 in either the Purkinje system (PS) or ventricular tissue; we used a geometrically detailed rabbit ventricular model with a representation of the PS [25] . Due to increased excitability in Purkinje fibres compared with ventricular cells [40] and the cable-like geometric structure of the PS [41] , we hypothesized that optical stimulation would elicit propagating responses at lower E e,thr values in the PS than in the ventricles. Selective ChR2 expression in distinct cell types has already been demonstrated in neuroscience [16] , [17] . Our simulation results would thus provide insight into whether the pursuit of optogenetic targeting of ventricular or PS cells would be worthwhile, which is important because cell-specific viral targeting remains a challenging process [42] . Ventricular models with GD of ChR2 in either the myocardium or PS were optically stimulated with illumination patterns designed to produce sinus-like activation sequences. In one model ( Fig. 6a ), patchy clusters of light-sensitive myocytes were located in 10 delivery sites corresponding to experimentally observed early activation sites [25] in regions of dense PS arborization. Each site contained both ChR2-expressing myocytes and non-photosensitive PS cells, as early activations emanate from Purkinje–myocardial junctions; the latter detail was important because it allowed us to use the same 10-site illumination setup to optically stimulate in the second model, which had gene-delivered ChR2 throughout the PS ( Fig. 6b ). Direct His bundle pacing by optical stimulation from a single optrode was also simulated in this second model ( Fig. 6c ). 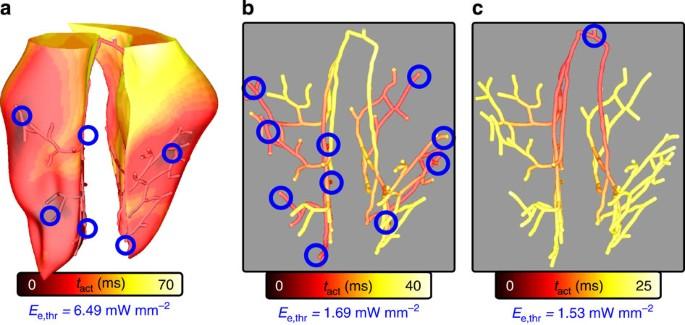Figure 6: Cell-specific optogenetic targeting in rabbit ventricles with Purkinje system. Each response shown here was elicited by applying 1.1 ×Ee,thrto the endocardial surface under each optrode for 2 ms att=0. In multioptrode models (a,b), all 10 delivery sites were illuminated simultaneously to achieve synchronous ventricular depolarization;Ee,thrwas the smallest value that initiated a propagating response when applied to each of the 10 sites independently. (a) Response to illumination of ChR2 delivery sites (blue) in regions of dense PS arborization (see text). Sites were hemispherical (2 mm diameter) with patchy GD of ChR2 in ventricular cells only (D=0.25,P=0.1). (b) Response to the same illumination pattern as in (a) but with GD optogenetic targeting of the PS only;Ee,thrwas 4.24 times lower compared with the model in (a). (c) Response to His bundle illumination for the same model as in (b);Ee,thrwas 3.84 times lower compared with the model in (a) and optical stimulation was only applied by 1 optrode compared with 10. Figure 6: Cell-specific optogenetic targeting in rabbit ventricles with Purkinje system. Each response shown here was elicited by applying 1.1 × E e,thr to the endocardial surface under each optrode for 2 ms at t =0. In multioptrode models ( a , b ), all 10 delivery sites were illuminated simultaneously to achieve synchronous ventricular depolarization; E e,thr was the smallest value that initiated a propagating response when applied to each of the 10 sites independently. ( a ) Response to illumination of ChR2 delivery sites (blue) in regions of dense PS arborization (see text). Sites were hemispherical (2 mm diameter) with patchy GD of ChR2 in ventricular cells only ( D =0.25, P =0.1). ( b ) Response to the same illumination pattern as in ( a ) but with GD optogenetic targeting of the PS only; E e,thr was 4.24 times lower compared with the model in ( a ). ( c ) Response to His bundle illumination for the same model as in ( b ); E e,thr was 3.84 times lower compared with the model in ( a ) and optical stimulation was only applied by 1 optrode compared with 10. Full size image As shown by activation maps for the ventricles and PS ( Fig. 6a ) or the PS only ( Fig. 6b,c ), the response to illumination was sinus-like in all cases; however, optical stimulation efficiency was dramatically higher for the model with GD of ChR2 to PS only, regardless of how it was illuminated. These differences could not be attributed to increased intrinsic PS excitability alone, as our simulations in single cells showed that E e,thr was only 1.60 times lower in individual Purkinje cells compared with ventricular myocytes (0.835 mW mm −2 and E e,thr =1.34 mW mm −2 , respectively, for 2 ms of illumination). Even when all ventricular target sites had consolidated instead of patchy spatial distribution, the E e,thr value (5.78 mW mm −2 ) was dramatically higher than for the photosensitive PS. Thus, in terms of stimulation efficiency, we conclude that the PS is a very attractive candidate for targeted, cell-specific optogenetic pacing. Optogenetic framework generalization Our newly developed framework is modular and can easily be combined with components that model other aspects of cardiac physiology. To illustrate this flexibility, we applied the framework to develop a light-sensitive electrophysiological model of the canine ventricles and PS, to which a cardiac mechanics component was added, as in previous studies [43] . Integration of electrical, mechanical and optogenetic modules is illustrated in Fig. 7a . Electromechanical simulation sinus rhythm and multi-site optical stimulation (as in Fig. 6a ) was performed using tools developed previously [44] . 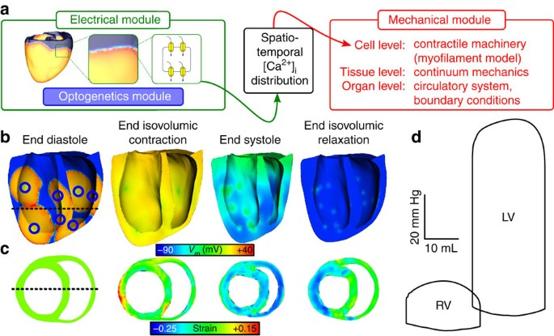Figure 7: Electromechanical response to optical stimulation in canine ventricles. (a) The electrical component (green), which encapsulates optogenetic framework model features (blue), is coupled with the mechanical component (red) by passing 3D intracellular [Ca2+] distribution from the ionic model to a cell-level myofilament model at each time step. (b,c) Long-axis membrane voltage (Vm) and short-axis strain profiles (unitless) during the cardiac cycle. Illumination delivered 12.8 mW mm−2to 10 ventricular ChR2 delivery sites (blue circles) for 10 ms att=0. Delivery sites were hemispherical (3 mm diameter) with consolidated CD expression. Dashed line in (b) shows position of slice in (c) and vice-versa. Strain was measured with respect to the end diastolic state. PS fibres were simulated but were not rendered graphically; regions of delayed repolarization due to long intrinsic PS action potential duration are visible in (b). (d) LV and RV pressure–volume loops for the photo-evoked response. These PV loops matched those for sinus rhythm very closely (cross correlation coefficientγ>0.9). The 10-site illumination pattern shown here resulted in a more vigorous contraction compared to optical pacing from the endocardial apex only (7.34% increase in stroke volume), due to increased depolarization synchrony (seeSupplementary Fig. S2). Figure 7: Electromechanical response to optical stimulation in canine ventricles. ( a ) The electrical component (green), which encapsulates optogenetic framework model features (blue), is coupled with the mechanical component (red) by passing 3D intracellular [Ca 2+ ] distribution from the ionic model to a cell-level myofilament model at each time step. ( b , c ) Long-axis membrane voltage ( V m ) and short-axis strain profiles (unitless) during the cardiac cycle. Illumination delivered 12.8 mW mm −2 to 10 ventricular ChR2 delivery sites (blue circles) for 10 ms at t =0. Delivery sites were hemispherical (3 mm diameter) with consolidated CD expression. Dashed line in ( b ) shows position of slice in ( c ) and vice-versa. Strain was measured with respect to the end diastolic state. PS fibres were simulated but were not rendered graphically; regions of delayed repolarization due to long intrinsic PS action potential duration are visible in ( b ). ( d ) LV and RV pressure–volume loops for the photo-evoked response. These PV loops matched those for sinus rhythm very closely (cross correlation coefficient γ >0.9). The 10-site illumination pattern shown here resulted in a more vigorous contraction compared to optical pacing from the endocardial apex only (7.34% increase in stroke volume), due to increased depolarization synchrony (see Supplementary Fig. S2 ). Full size image Figures 7b and c show the spatiotemporal sequence of V m propagation and strain development during a heartbeat elicited by sinus activation-like optical pacing. Initial excitations for optical stimulation differed from those during sinus rhythm because delivery sites were illuminated simultaneously, so the detailed spatiotemporal order of PS excitation was not replicated. The hemodynamic responses in the two models were near identical (see pressure–volume loops in Fig. 7d ). These simulations demonstrate the utility of the combined optogenetic–electromechanics model, which could be used to design and optimize novel, light-based therapies for treating contractile dyssynchrony in the heart. In this study, we developed a comprehensive framework for incorporating optogenetic phenomena in detailed multiscale simulations of cardiac electrophysiology. Optogenetic capabilities were developed at each model scale: at the cell level, we modelled photokinetics of the light-sensitive ChR2 channel and represented ChR2 delivery either directly to myocytes (GD) or via donor cells (CD); at the tissue level, we modelled realistic heterogeneous spatial distribution of ChR2-expressing cells; and, at the organ level, we incorporated a physically accurate model for illuminating light-sensitive tissue. We then applied the newly developed framework in two case studies that aimed to illustrate its capability: first, we showed that spatial distribution of light-sensitive cells affected optical stimulation efficiency differently depending on ChR2 delivery mode; second, we showed that optical stimulation was more efficient when cell-specific optogenetic targeting was used to express ChR2 in Purkinje cells compared with ventricular myocytes. Finally, we combined the optogenetic electrophysiological model with a cardiac mechanics component to demonstrate the modularity of the framework and highlight the ease of integrating optogenetics in multiscale, multiphysics heart models of arbitrary complexity. Here, we discuss results presented in our study and potential future applications of our framework; in the Supplementary Discussion section, we elaborate on the significance of multiscale optogenetic modelling capabilities and the versatility of the framework, we discuss the feasibility and energy efficiency of optical stimulation and we propose strategies for validating the results of this study in vitro . Our findings indicate that ChR2 delivery mode and light-sensitive cell spatial distribution have important roles in determining the threshold irradiance for optical stimulation. In the context of simulated ChR2 delivery by injection in the intact heart, ChR2-rich donor cells (CD) with low density and high patchiness are associated with lower E e,thr values than the same distributions of ChR2-expressing myocytes (GD), indicating higher efficiency. This is due to the fact that patchy distributions of cell-delivered ChR2 maximize the interface between electrical sources (donor cells) and sinks (myocytes at rest) during the excitation phase. This result is relevant to practical optogenetic therapy because ChR2-expressing cells can die or migrate away from the original delivery site over time, leading to decreased density and increased patchiness; our model indicates that optical stimulation is more likely to remain viable in spite of such changes if ChR2 is delivered via donor cells (CD) as opposed to viral transfection (GD), which is a hypothesis that could be validated experimentally. Our framework provides an ideal platform for further analysis of this important problem because it accounts for all major factors that might affect optical stimulation efficiency. We also show that if a PS-specific promoter can be developed to achieve targeted gene delivery with high expression density, optical stimulation can be used to elicit sinus-like paced activations at low irradiances. Purkinje fibres are more easily excited than well-coupled ventricular myocytes due to differences in membrane kinetics [40] (cell-level) and dramatically reduced source–sink mismatch due to network geometry [45] (tissue-level). Moreover, as PS fibres tend to run along or just beneath the endocardial surface, light attenuation does not have such a dramatic effect. Direct His bundle pacing by conventional electrical stimulation can overcome bundle branch block and restore synchrony in certain cardiac resynchronization therapy candidates, but pure His capture is difficult to attain and energy requirements are very high [46] ; our findings suggest that both of these shortcomings—lack of selectivity and low energy efficiency—could be mitigated by applying optogenetics to facilitate direct optical His bundle pacing. Selective inscription of light sensitivity in specific cell types has already been demonstrated in neuroscience [16] and should be possible in the PS. That said, the process of engineering a viral vector to accurately and efficiently target a particular cell type without toxic side effects is both costly and difficult [42] . Our simulations of optogenetic targeting of Purkinje cells show how the framework can be leveraged to rapidly and accurately assess such high-risk, high-reward therapeutic strategies before the investment of considerable resources and effort in wet lab. Although our framework integrates all presently available information regarding cardiac optogenetics, there are still numerous unknown physiological factors. As such, we are cognizant of the fact that the above conclusions must be subjected to validation in vitro and have indicated future directions accordingly (see: Supplementary Discussion ). This inherent uncertainty also reaffirms the importance of our framework’s modularity—as new details become available, they can be integrated at the appropriate levels of model hierarchy and new and more accurate simulations can be run. As the framework continues to be expanded, it can be used to explore optogenetics-based solutions to many open problems in cardiac electrophysiology. For example, early investigation of multipulse pacing for arrhythmia termination suggested that PS stimulation was an important determinant of therapy success [47] but subsequent studies have not explored this connection in depth. Direct optical stimulation of the PS only (and not surrounding myocardium) could help elucidate this complex matter and defibrillation by illumination may prove to be a plausible option. Sustained low-amplitude illumination of depolarizing or hyperpolarizing opsins [18] could be used to dynamically modulate the firing rate of autorhythmic myocytes [22] or to add pacemaker functionality to quiescent myocytes [21] . Weak hyperpolarizing optical stimuli could also be used to suppress ectopic activity near the endocardium, where the safety factor for propagation is elevated [48] and attenuation does not limit the ability to optically modulate V m . A similar approach using an excitatory opsin could be used to increase the heart’s propensity for triggered activity, providing a valuable diagnostic tool for identifying sites with the highest likelihood of producing ectopic beats. Another exciting possibility is the use of ChR2 and other opsins to shape AP repolarization [17] . Optogenetics could be used as a novel therapeutic approach to shorten or lengthen AP duration in a regionally heterogeneous manner. This could be especially useful in the treatment of long and short QT syndromes, heart failure and abnormal ventricular wall motion, as changes in transmural dispersion of repolarization are thought to catalyse arrhythmogenesis in all of these disorders [49] , [50] , [51] , [52] . Our computational framework for simulating cardiac optogenetics is a predictive tool that will drive hypothesis development and provide a platform for detailed mechanistic enquiry. The modelling methodologies specified here can be implemented in any computational cardiology software and used to accurately simulate opsin delivery and optical stimulation in cardiac models of arbitrary complexity and for a variety of species. As the field of cardiac optogenetics matures, in silico tools will provide insight and guidance that could help anticipate pitfalls, minimize expensive and time-consuming wet lab experiments and fully characterize the underlying mechanisms of therapeutic techniques. Light-sensitive current model For this study, we developed a model of ChR2 current ( I ChR2 ) based on the four-state photocycle [29] . This model incorporated closed and open states for light- and dark-adapted operating modes. A ChR2 parameter set was generated from previously published values to produce currents qualitatively consistent with those obtained from whole-cell patch-clamp recordings. Some modifications to the original four-state model [29] were included; that is, the ChR2 channel activation rate was captured using a time- and light-dependent state variable p as in Talathi et al. [53] , and some parameters were adopted from Grossman et al. [54] (see Supplementary Table S1 ). In addition to light sensitivity, our model incorporated a simplified linear current–voltage relationship and was scaled via the maximum conductance ( g ChR2 =2 mS cm −2 ) so that peak current qualitatively matched experimental data from whole-cell patch clamp experiments in a stable HEK cell line expressing ChR2–H134R (a ChR2 mutant with enhanced current), which has been described previously [21] . The governing I ChR2 equation was: where γ =0.1 was the conductance ratio between open states ( O 2 : O 1 ), g ChR2 =2 mS cm −2 was the maximal channel conductance and E ChR2 =0 mW was the reversal potential. Although open ChR2 channels approached an E e -dependent equilibrium between dark- and light-adapted modes; closed channels recovered very slowly from light adaptation ( τ =250 ms) compared with other transition kinetics. A complete listing of I model equations and parameters is provided in Supplementary Table S1 . Donor cell model for CD mode Instead of explicitly representing HEK-ChR2 cells, we modelled light-sensitive donor cells using an electrically passive membrane model with I ChR2 . HEK-ChR2 cells do have other low-conductance channels, but these have not been characterized in detail and contribute negligibly to optical excitability [21] ; thus, our model includes the key characteristics of donor cells (compared with normal myocytes)—light sensitivity and the lack of an active response. The electrically passive membrane model used for donor cells in CD mode was given by: where g PASV =14 μS cm −2 was the specific membrane conductivity and V rest =−40 mV was the resting potential. These properties were based on measurements from HEK cells [21] , [55] . Like all excitable cells modelled, specific membrane capacitance was assumed to be 1 μF cm −2 . In donor cell–myocyte tandem pairs, the two membrane models were coupled by a 500 MΩ resistance. In organ-scale simulations, donor cell clusters (CD) were modelled with reduced, isotropic conductivity: σ donor =0.2 × σ iL , where σ iL is the intracellular conductivity along the myocyte axis. We made this choice based on reported properties of HEK cell clusters, which lack the fibre-like arrangement of heart tissue and have diminished cell–cell coupling [21] . Light-sensitive cell distribution algorithm Each simulated ChR2 delivery site was described by a sphere of radius ( r ) surrounding a node ( n ) on the endocardial surface of the finite element mesh. We began by building a list of N mesh elements completely contained within the distance r from node n . Then, elements were tagged as light-sensitive one by one until the number of tagged elements was ≥ D × N , where D is the density parameter. The process of choosing which elements to tag was governed by a stochastic distribution algorithm developed for use in two-dimensional (2D) cardiac cell monolayers [36] . The process of extending this algorithm into 3D was straightforward: rather than examining shared edges to determine the neighbourhood around each cluster, we identified shared faces and applied the distribution process described in the original paper. Briefly, for each new light-sensitive element, the probability of starting a new cluster instead of adding to an existing one was P , the patchiness parameter. One important constraint was necessitated by the 2D to 3D extension—seed elements for new clusters were always chosen from the subset of elements touching the endocardial boundary; we chose this constraint because transfected and/or donor cells tend to congregate near the injection site [34] , [35] . Supplementary Fig. S3 shows an example of simulated ChR2 delivery in a representative 2D schematic and summarizes how node- and element-level optogenetic properties are assigned for GD and CD of ChR2. Simulation details We ran monodomain simulations of electrical activity using the CARP software package [33] , [56] ; simulation results were visualized using Dr Edward Vigmond’s meshalyzer tool. Ventricular cell membrane kinetics in the human model were simulated according to the formulation developed by ten Tusscher and Panfilov [31] as modified by Moreno et al. [24] In the rabbit model, we used the Mahajan–Shiferaw AP model in the ventricles [57] and the Aslanidi–Sleiman AP model in Purkinje fibres [58] ; PS–myocardial junction dynamics were simulated using a previously validated model [59] . Other relevant model parameters for the human and rabbit electrophysiological models are provided in Supplementary Tables S2 and S3 , respectively. How to cite this article: Boyle, P. M. et al. A comprehensive multiscale framework for simulating optogenetics in the heart. Nat. Commun. 4:2370 doi: 10.1038/ncomms3370 (2013).